Direct measurement of osmotic pressure via adaptive confinement of quasi hard disc colloids Confining a system in a small volume profoundly alters its behaviour. Hitherto, attention has focused on static confinement where the confining wall is fixed such as in porous media. However, adaptive confinement where the wall responds to the interior has clear relevance in biological systems. Here we investigate this phenomenon with a colloidal system of quasi hard discs confined by a ring of particles trapped in holographic optical tweezers, which form a flexible elastic wall. This elasticity leads to quasi-isobaric conditions within the confined region. By measuring the displacement of the tweezed particles, we obtain the radial osmotic pressure. We further find a novel bistable state of a hexagonal structure and concentrically layered fluid mimicking the shape of the confinement. The hexagonal configurations are found at lower pressure than those of the fluid, thus the bistability is driven by the higher entropy of disordered arrangements, unlike bulk hard systems. Phenomena induced by confinement include decoupled dynamics parallel and perpendicular to boundaries, the adoption of structures mimicking the confining geometry and the formation of novel phases. Such behaviour is found in a broad range of systems including simple [1] , [2] , [3] , [4] and molecular [5] , [6] liquids, colloidal and nanoparticle suspensions [7] , [8] , [9] , [10] , [11] , [12] and granular materials [13] . As a result, confinement offers new routes to self-assembly and control of reaction rates and pathways [4] , [14] , [15] , [16] . Underlying the impact of confinement upon a system, leading to changes in structure, dynamics and phase behaviour, is its effect upon the free energy [17] , which can be accurately determined for model systems such as we employ here. Combined with direct comparison to bulk behaviour [18] , [19] , [20] , such calculations enable an understanding of the effects of confinement. By emphasizing adaptive confinement, we open the possibility to use colloids as basic models of biological systems such as cell walls. Our system comprises a suspension of polystyrene colloids in a water–ethanol mixture, in which 27 particles of diameter σ =5 μm are held by holographic optical tweezers (HOT) [21] in a ring configuration ( Fig. 1 ). These ring particles thus form a flexible ‘membrane’ that can adapt to the interior. The colloids are restricted to quasi-two-dimensions (2D) by gravity, thus the ring, or corral, confines a population of up to N =49 particles. We express the interior population in terms of the effective area fraction where σ eff is the Barker–Henderson effective hard sphere diameter [22] accounting for electrostatic interactions between the colloids and ‹ A Vor › is the average area accessible to an interior particle. Further details are provided in the Methods. Coordinates of both interior and membrane particles are obtained throughout the experiment. We compare our experimental results with 2D Monte-Carlo simulations of a hard disc system that is similarly confined. In our study of quasi hard discs, adaptive confinement introduces two main effects. First, by measuring displacements of the membrane particles we directly obtain the osmotic pressure in the interior. Thus, our system marks a departure from the constant-volume ensemble characteristic of soft matter, as the fluctuating membrane exerts a pressure on the interior creating instead a quasi-isobaric ensemble. Second, the combined experimental and simulation approach reveals that adaptive confinement enables hexagonal ordering reminiscent of the bulk [18] , [19] , [20] , leading to a bistability between this structure and a layered fluid characteristic of similarly confined hard wall systems [1] , [2] , [7] . 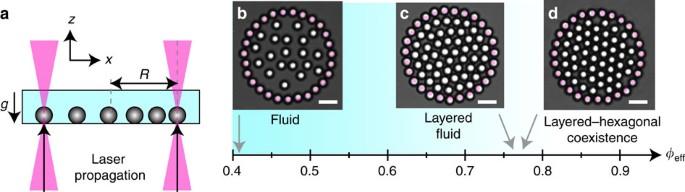Figure 1: Colloidal corral system overview. (a) Schematic showing side view of experimental system defined by corral radiusR. (b–d) Phase diagram as a function of effective area fraction,φeff, with images of fluid, layered fluid and hexagonal structures. Scale bars represent 10 μm. Note that the images of the layered fluid (c) and hexagonal structure (d) both have interior populationN=48. Pink circles in (b–d) indicate positions of optical traps. Figure 1: Colloidal corral system overview. ( a ) Schematic showing side view of experimental system defined by corral radius R . ( b – d ) Phase diagram as a function of effective area fraction, φ eff , with images of fluid, layered fluid and hexagonal structures. Scale bars represent 10 μm. Note that the images of the layered fluid ( c ) and hexagonal structure ( d ) both have interior population N =48. Pink circles in ( b – d ) indicate positions of optical traps. Full size image Phase behaviour and structure The phase diagram of the system is shown in Fig. 1b–d . By increasing the corral population a qualitative change in structure is observed. At low density, the interior structure is fluid-like ( Fig. 1b ), but upon increasing the population, a concentrically layered structure consisting of rings of particles mimicking the symmetry of the confining boundary becomes evident ( Fig. 1c ). In our experiments, we sometimes find hexagonal ordering for effective area fraction φ eff ≳ 0.77 ( Fig. 1d ). The degree of local hexagonal ordering is quantified using the bond-orientational order parameter, where z j is the co-ordination number as defined by a Voronoi construction and is the angle made by the bond between particle j and its m th neighbour and a reference axis. For perfect hexagonal ordering, ψ 6 =1, whereas totally disordered systems have ψ 6 =0. We consider ψ 6 >0.775 to represent a hexagonal structure. As the hexatic transition in bulk hard discs has been identified in the range 0.70≤ φ ≤0.716 (ref. 20 ), we assume our system explores the kind of configurations a bulk system at the same area fraction would exhibit. Owing to curvature, hexagonal ordering is suppressed in the layer of particles by the wall. However, upon sufficient lowering of the spring constant in the optical traps by reducing the laser power, the adaptivity of the corral is enhanced. Under these conditions complete hexagonal ordering may be possible. In simulation, hexagonal ordering is most strongly suppressed at high spring constant, and is enhanced as the spring constant is reduced ( Supplementary Fig. S1 ). Thus, local hexagonal ordering imposed by packing constraints competes with concentric layering imposed by the boundary shape. Such hexagonal structure has not, to the best of our knowledge, been reported for systems of comparable size confined by hard boundaries. We argue that this structure, which more closely resembles the bulk than the confining geometry, is made possible by the adaptive confinement. Wall roughness on the particle lengthscale has been shown to inhibit particle layering [2] and although the walls of this system are indeed rough, the roughness is naturally commensurate with the particle size and interparticle separation. If the circular boundary were ‘flattened’, removing the wall curvature, the regular spacing of the optically trapped particles would promote hexagonal ordering. However, the curvature of the boundary is incommensurate with hexagonal order, suppressing ψ 6 in its immediate vicinity to , ( Supplementary Fig. S2 ) indicating that wall roughness is not the source of the observed locally hexagonal structure but that it is made possible by the adaptive confinement that can be distorted. We explore these competing structures further in Fig. 2a where ψ 6 is plotted as a function of packing fraction. There is a general trend of increasing ψ 6 with area fraction for φ eff <0.77. Concentrically layered structures such as that shown in Fig. 1c for N =44 have ψ 6 in the range 0.6< ψ 6 ≲ 0.75. In our experiments, at high packing fractions, a distribution of populations with high and low ψ 6 are found. These correspond to hexagonal and layered fluid structures respectively. For hard systems in general, we associate entropically driven ordering with an increase packing, and hard discs are no exception [20] . 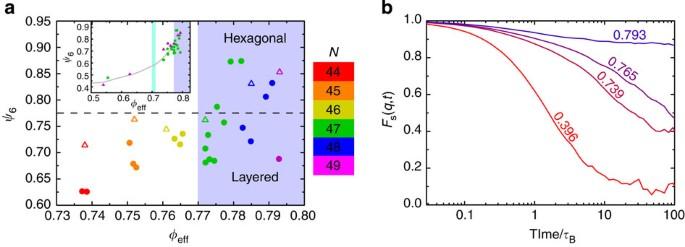Figure 2: Structure and dynamics in adaptive confinement. (a) Average local hexagonal order parameterψ6as a function of effective area fraction. Horizontal dashed line demarcates hexagonal structures (ψ6>0.775) from layered structures (ψ6≤0.775). Circles are experimental data, open triangles are simulation. Blue shaded region represents densities at which concentrically layered structures compete with locally hexagonal structures. Points are coloured by corral population,N. Inset includes low-density data in the bulk fluid regime. Fluid-hexatic phase coexistence in the bulk20is indicated by the turquoise region. Line is to guide the eye. (b) Experimental self ISF,FS(q,t), at different effective area fractions,φeff. Lines labelled withφeff. The wavevectorq=2π/σeffis taken close to the main peak of the static structure factor. Figure 2: Structure and dynamics in adaptive confinement. ( a ) Average local hexagonal order parameter ψ 6 as a function of effective area fraction. Horizontal dashed line demarcates hexagonal structures ( ψ 6 >0.775) from layered structures ( ψ 6 ≤0.775). Circles are experimental data, open triangles are simulation. Blue shaded region represents densities at which concentrically layered structures compete with locally hexagonal structures. Points are coloured by corral population, N . Inset includes low-density data in the bulk fluid regime. Fluid-hexatic phase coexistence in the bulk [20] is indicated by the turquoise region. Line is to guide the eye. ( b ) Experimental self ISF, F S ( q , t ), at different effective area fractions, φ eff . Lines labelled with φ eff . The wavevector q =2π/σ eff is taken close to the main peak of the static structure factor. Full size image Before turning to the cause of this apparent degeneracy in ψ 6 at high area fraction, we address its connection with ergodicity. To investigate the dynamics, we calculate the self intermediate scattering function (ISF) F S ( q , t )=‹| e iq [ r ( t + t ′)— r ( t ′)] |› where the angle brackets indicate averaging over particles and t ′ and the wavevector . The resulting ISFs are plotted in Fig. 2b . For φ eff ≳ 0.75, the ISF does not decay on the experimental timescale (2.03 × 10 4 s or 290 Brownian diffusion times, τ B ), indicating that the system does not reach equilibrium. Thus, it is possible that the amorphous structures could be metastable to hexagonal configurations or even vice versa . As we shall see however, this degeneracy is in fact a manifestation of a bistable state found at high density. By contrast, our simulations do reach equilibrium, as shown in Supplementary Fig. S3 . Thus we find one value of ψ 6 for each φ eff in Fig. 2a . In order to observe full decay of the experimental ISFs at all area fractions considered, much longer experiments would be required. We estimate that an experimental duration of ~200 h is required for full equilibration of all experimental samples. Additionally, ergodicity may be recovered through a reduction in boundary stiffness, via reduction in φ eff , as a softer boundary allows the system to expand. We estimate that if the trap stiffness falls to ~ 0.45; of its experimental value then the N =49 particle system would relax on the experimental timescale. Measurement of pressure Owing to the elasticity of the confinement, densely populated corrals have a radius that is, on average, larger than that of the unpopulated corral. The confining boundary is ‘stretched’ by the interior population, displacing the wall particles from their optically defined energy minima at R 0 ≈4.32 σ eff . For small deformations of the corral, we assume each trap creates an identical Hookean restoring force around each particle in the ring (see Methods and Supplementary Fig. S4 ). By measuring the expansion of the corral with respect to its unpopulated size, we directly obtain the osmotic pressure of our system. The Hookean restoring force on each trapped particle is F =−λ( R – R 0 ). We average over all 27 trapped particles when calculating R . That the force experienced by each trapped particle can be treated as identical is important—it indicates the system is quasi-isobaric. 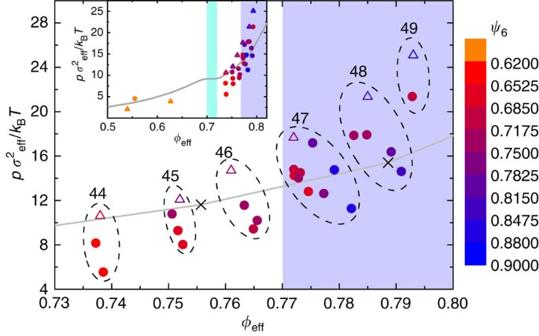Figure 3: Pressure measurement. Dimensionless radial pressure as a function of area fraction for both experiment (filled circles) and Monte-Carlo simulation (open triangles). Symbols are grouped inside dashed lines indicating the corral population,N, they represent and are coloured based on the average value ofψ6of particles non-adjacent to the corral wall with red points indicating lowψ6and blue points indicating highψ6. Black crosses joined by grey lines are data from bulk hard disc simulations24. Inset includes low-density data in the bulk fluid regime. Fluid-hexatic phase coexistence in the bulk20is indicated by the turquoise region. Grey line indicates bulk pressure for the fluid23and the solid24. Shaded blue regions denote area fractions for which bistable behaviour is observed. The pressure is calculated as Figure 3 shows the dimensionless time-averaged radial pressure calculated using Equation 1 for experimental and simulated corral systems in the range 0.50≤ φ eff ≤0.8. For state points where bulk hard discs are fluid ( φ eff ≤0.70), we find good agreement between pressure measurements of our confined system and bulk values [23] . The symbols are coloured based on the value of ψ 6 plotted in Fig. 2 , with red indicating low ψ 6 (concentric layering) and blue indicating high ψ 6 (local hexagonal ordering). Figure 3 reveals the interplay between pressure and ordering: for a given population, higher ψ 6 samples in general exhibit lower pressures and higher area fractions. Figure 3: Pressure measurement. Dimensionless radial pressure as a function of area fraction for both experiment (filled circles) and Monte-Carlo simulation (open triangles). Symbols are grouped inside dashed lines indicating the corral population, N , they represent and are coloured based on the average value of ψ 6 of particles non-adjacent to the corral wall with red points indicating low ψ 6 and blue points indicating high ψ 6 . Black crosses joined by grey lines are data from bulk hard disc simulations [24] . Inset includes low-density data in the bulk fluid regime. Fluid-hexatic phase coexistence in the bulk [20] is indicated by the turquoise region. Grey line indicates bulk pressure for the fluid [23] and the solid [24] . Shaded blue regions denote area fractions for which bistable behaviour is observed. Full size image At high packings ( φ ≳ 0.77), the experimental system does not reach equilibrium. As our measurements of pressure are mechanical, we can measure p for such non-equilibrium state points ( Fig. 2b ). However, because phase space is not fully sampled, each experiment gives a different pressure value, resulting in a range of observed pressure for a given interior population. Conversely, because our simulations reach equilibrium, a single value is found for the pressure. Our system exhibits a departure from bulk behaviour [24] for φ ≳ 0.77, a similar packing fraction to that at which the system starts to visit hexagonal configurations. We assume that such a deviation is due to confinement. Structural bistability Although the highly ordered hexagonal structures feature a lowering in pressure, which in bulk systems indicates a reduction in free energy, here we find these coexist with higher pressure disordered layered fluid structures. We find transitions between both structures, accompanied by changes in area fraction and ψ 6 . Examples are given in Fig. 4 , which shows the time evolution of the instantaneous area fraction, pressure, ψ 6 and mean-squared particle displacement for a sample of population N =47. The system initially undergoes a transition from high to low area fraction and high to low ψ 6 . A structure similar to the original is recovered between 140–170τ B . These transitions are indicated by the dashed lines in Fig. 4a–d and occur over a time interval of ~10τ B and 30τ B , respectively. Figure 5a shows the particle rearrangements in the second transition time interval (purple data in Fig. 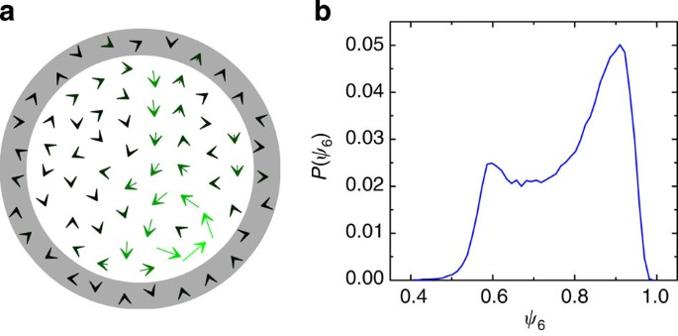Figure 5: Dynamical heterogeneity and structural bistability. (a) Displacement of particles in transition period around 140–170τBinFig. 4. Magnitude of displacement is indicated by the length and colour of each arrow. Arrows in grey ring correspond to particles in optical traps forming the confining wall. (b) Distribution ofψ6from simulated configurations atN=47. 4a–d at 140–170τ B ), resulting in this increase in volume fraction and decrease in pressure. 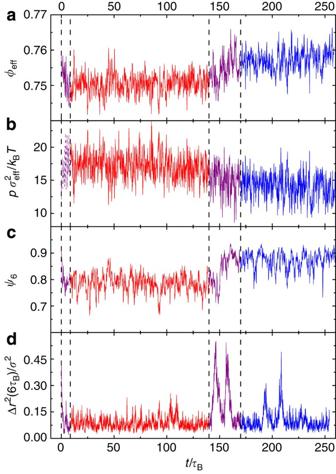A cooperative rearrangement of particles, strongly localized in time, results in a structural change in the system, allowing the boundary to contract. Figure 4: Experimentally observed structural transitions. Time evolution of (a) instantaneous effective area fraction (b) pressure (c)ψ6and (d) mean squared particle displacement over a timescale of 6τBfor a single sample of populationN=47. Transitions occur, initially down from a highψ6configuration att=0 and later from a lowφeff, high-pressure configuration to one at higherφeffand lower pressure. Transition intervals are indicated by vertical dashed lines. Figure 4: Experimentally observed structural transitions. Time evolution of ( a ) instantaneous effective area fraction ( b ) pressure ( c ) ψ 6 and ( d ) mean squared particle displacement over a timescale of 6 τ B for a single sample of population N =47. Transitions occur, initially down from a high ψ 6 configuration at t =0 and later from a low φ eff , high-pressure configuration to one at higher φ eff and lower pressure. Transition intervals are indicated by vertical dashed lines. Full size image Figure 5: Dynamical heterogeneity and structural bistability. ( a ) Displacement of particles in transition period around 140–170 τ B in Fig. 4 . Magnitude of displacement is indicated by the length and colour of each arrow. Arrows in grey ring correspond to particles in optical traps forming the confining wall. ( b ) Distribution of ψ 6 from simulated configurations at N =47. Full size image On the experimental timescale, such cooperative rearrangements are rare. Dynamically, the system is characterized by long periods of low particle mobility at different area fraction (or pressure) separated by short rearrangement intervals of higher particle mobility (Δ r 2 >0.3 σ 2 ), during which a subset of the system undergoes cooperative, neighbour-changing motion, as shown in Fig. 4d . Such isolated events are the mechanism by which the system relaxes. Thus we find temporal dynamic heterogeneity. In other words, rearrangements correspond to active periods interspersed with inactive periods. Such temporally heterogeneous dynamics between inactive and active periods have been related to the glass transition [25] . Plots such as that shown in Fig. 5a allow the visualization of the size and shape of co-operatively rearranging regions, which yields detailed information about the nature of slow dynamics in confinement. Data such as those in Fig. 4 indicate that the system undergoes transitions between two structures, one of high order and low pressure and one of high pressure and low order. To test this hypothesis, we plot the probability distribution of ψ 6 as obtained from Monte-Carlo simulation in Fig. 5b . Indeed the behaviour is consistent with structural bistability in that two peaks, one corresponding to each structure, are found. A similar plot obtained from experimental data is shown in Supplementary Fig. S5 , although our experiments do not reach full equilibrium at these high area fractions. Figure 5b provides strong evidence that the adaptive confinement induces a bistability in these assemblies of hard discs between a layered fluid (with high pressure and low order) and a hexagonal system (with low pressure and high order). This contrasts strongly with phase coexistence in bulk systems, where coexistence of a fluid and a crystal occurs at a single pressure but at different volumes (or equivalently, areas). Pressure and area are coupled in our system and therefore the two coexisting structures have distinct areas and pressures. At first sight, the emergence of a hexagonal structure at high density seems reminiscent of bulk hard discs. However, our adaptive confinement introduces a potential energy to the system. Indeed, that the hexagonal structure resides at lower pressure and higher order would suggest that it should be strongly favoured. That we find the system in layered fluid configurations at all indicates that more is at play than energy. This leaves entropy, and in fact there are fewer configurations accessible to the hexagonal structure. This is because free volume is expended in the ‘voids’ close to the walls in Fig. 1d . Thus, because the layered fluid fits the cavity better than the hexagonal configuration, it is entropically favored, in contrast to the case of bulk hard discs. Further evidence for this scenario is provided by the suppression of hexatic ordering relative to the bulk, where it is found for φ ≥0.716 (ref. 20 ). Here we find hexatic ordering only for φ eff ≥0.77. This suppression results from the entropic loss associated with the hexatic ordering. The prescence of voids adjacent to the boundary in hexagonally ordered systems is also indicated in Supplementary Fig. S6 , where the local area fraction is found to decrease towards the boundary of the corral for both concentrically layered and locally hexagonal configurations. This effect is stronger in the case of the hexagonally ordered system, where the local area fraction adjacent to the boundary is suppressed by ~3% relative to the average. In the layered fluid this suppression is only half as strong, with local area fraction ~1.5% lower than the average. As the observed structural bistability is dependent upon the adaptivity of the boundary, it is feasible that controlled modification of the wall can induce transitions between layered and hexagonal structures. The corral wall is defined by its size, shape and stiffness. Altering any one of these in situ can potentially drive the confined system from one structure to another. For instance, a hexagonal configuration can be ‘melted’ by increasing the diameter of the confining ring. Similarly, hexagonal configurations can be favoured by altering the shape of the confining boundary—the extreme case of this being confinement by a hexagonal wall ( Supplementary Fig. S7 ). Furthermore, as noted above, stiffer boundaries inhibit hexagonal ordering ( Supplementary Fig. S1 ), which indicates that increasing optical trap strength is capable of driving a locally hexagonal configuration into a concentrically layered configuration and vice versa. A confined model experimental system of quasi hard discs is introduced with a ring of particles held in HOT. Monte-Carlo computer simulations show that the system is well described as hard discs confined by particles in harmonic potentials. We demonstrate that measuring the expansion of the optically defined confining boundary due to interior particles enables direct measurement of the radial osmotic pressure of the confined system. As the confining wall adapts to the interior, many more configurations can be accessed than in conventional static confinement. In particular, we find hexagonal ordering reminiscent of the bulk, which competes with concentric layering echoing the ring of trapped particles. Furthermore, for a given number of interior particles, the system is quasi-isobaric, enabling transitions between these two structures—a bistable state. Unlike the case for bulk systems, here the configurational entropy of the hexagonal structure is lower than that of the fluid, because it is incommensurate with the circular boundary. It would be interesting to carry out microscopic density functional calculations for hard disks in order to predict the structural and dynamical collective behaviour of the confined systems [26] . Our system is ideal for studying the basic properties of adaptive confinement and can readily be generalized to three dimensions (3D). This would enable the osmotic pressure measurements to be applied to other systems, including active matter such as driven colloids [27] and bacteria. By constructing a corral around a cell and varying the salt concentration, our technique might even enable the turgor pressure to be directly determined. Moreover, as ensembles of rigid non-spherical particles are used as an approximation to the cytoplasm [28] , our approach could even model some properties of cells. Finally, with a suitable choice of geometry, for example a fixed cylinder with a 2D tweezed array, realization of nanoscale Brownian pistons is now feasible, which would enable direct tests of basic thermodynamic behaviour such as compression. Sample details The experimental system consists of polystyrene colloids of diameter σ =5.0 μm with a polydispersity of 2%, suspended in a water–ethanol mixture at a ratio of 3:1 by weight. The Debye length in our experimental samples is estimated by matching the Barker–Henderson effective hard sphere diameter [22] to the simulated hard disc diameter that best reproduces experimental behaviour. This results in a Debye length of κ −1 ≈25 nm, which is consistent with the experimental conditions. We assume the effective colloid charge Z eff is given by Z eff λ B /σ~6. This leads to a Barker–Henderson effective hard sphere diameter σ eff =5.08 μm. The density mismatch between the particles and the solvent is such that their gravitational length is l g / σ eff =0.015(1), which results in fast sedimentation of suspended particles and the formation of a quasi-2D monolayer adjacent to a glass coverslip substrate. This coverslip is made hydrophobic by treatment with Gelest Glassclad 18 to prevent particle adhesion. The Brownian time, τ B , is determined empirically by measuring the mean-squared displacement in a dilute system. We define Brownian time as the average time needed to diffuse a distance of one particle radius. For our experimental conditions we measure a Brownian time of τ B ≈70.2 s. Holographic optical tweezers The HOT apparatus consists of an ytterbium fibre laser of wavelength 1,064 nm modulated by a computer-addressed liquid crystal on a silicon spatial light modulator (Holoeye PLUTO-NIR) capable of applying phase shifts of up to 2π to laser light reflected from each of its 1,920 × 1,080 pixels. The application of superposed phase gratings to the SLM modulates the incident beam such that it can form arbitrary arrays of optical traps [21] . The HOT apparatus is controlled using LabVIEW software adapted from that developed by the Glasgow University Optics Group [29] . Optical trapping is integrated into an inverted microscope (Zeiss Axiovert 200) and facilitated by a high numerical aperture objective (Zeiss Plan-Neofluar × 100 magnification). This same objective images the sample to a charged coupled device camera (Allied Vision Technologies Dolphin F-145B), which relays sample images to the computer. The colloidal corral As shown in Fig. 1 , 27 particles are positioned using HOT forming the adaptive corral boundary. These traps are well-approximated by parabolae with spring constant λ =302(2) . This spring constant is determined by measuring the probability distribution of radial coordinates for particles forming the boundary in the absence of a confined population. By assuming this radius is Boltzmann-distributed the optical potential is extracted and fit with the parabolic form characteristic of a Hookean spring (see Supplementary Fig. S2 ). As we find a good degree of uniformity in the strength of our optical traps, we consider an effective corral potential described by a single spring constant, rather than extracting individual spring constants for each of our 27 optical traps. Variations in the radial spring constant for individual optical traps are a few percent of the value of the effective spring constant. It is integral to this work that the confined particles are unaffected by the light field used to create the circular boundary. The light field due to the 27 optical traps is assessed by imaging the laser light reflected from a glass–air interface at maximum camera gain. Supplementary Fig. S8a shows a single image of the light field in which the 27 optical traps are clearly visible. If the intensity of each pixel is summed over a sequence of images one obtains the composite image in Supplementary Fig. S8b , in which background noise is suppressed. It is clear from these high-gain images of the light field that the interior region is free from unwanted optical influence. Experimental data are acquired for up to 6 h at 0.5 frames per second. Particle trajectories are extracted [30] for corral populations N ≤49 corresponding to area fractions φ eff <0.8. Area fraction is estimated from experimental data by considering the Voronoi decomposition of the particle coordinates for each frame. The particles forming the confining boundary are neglected—only the Voronoi cells of the interior population are considered. In a given frame, the instantaneous area fraction is defined using the circular cross-sectional area of a particle (assuming particles are monodisperse) and the average Voronoi cell area (or the average area per particle). For densely populated corrals this gives a good estimate of the area fraction; however, at low densities, as the Voronoi polygons of the particles forming the confining walls penetrate further into the corral interior, this method may over-estimate the area fraction. Unless a distinct transition is observed in the course of an experiment, the area fraction is taken to be the time average of the instantaneous area fraction. Data exhibiting a transition is split into pre- and post-transition sequences and thereafter treated as distinct experiments. Monte-Carlo simulation Monte-Carlo simulations reproduce the experiments. N hard discs are placed in a circular region enclosed by 27 additional discs. To reproduce the confining effect of the optical tweezers, each of these 27 discs lies in a parabolic potential energy well of stiffness λ =302 as found by fitting experimental data. The experimental system is quasi-2D and the electrostatic charge leads to some softness in the interparticle interactions. Even without these considerations, in 2D the accuracy to which φ eff can be determined is ≳ 4% (ref. 31 ). The effect of interactions complicates the situation [32] . Here we treat R 0 as a fit parameter, with 4.30≤ R 0 ≤4.44 and find best agreement with R 0 =4.32. We perform five independent runs for each N using 10 7 Monte Carlo sweeps to equilibrate the system. Although considerable fluctuations are seen between different configurations, at a given state point no significant changes in φ , ψ 6 or pressure are observed between any of our runs, so we assume that the system is equilibrated. Supplementary Fig. S3 presents further evidence of ergodicity in simulation. Confirmation that the simulations of 2D hard discs are a good approximation to our experimental system is provided in Supplementary Fig. S9 , where we explicitly include the effect of gravity to form a quasi-monolayer in a 3D system and model electrostatic interactions via a Yukawa potential. How to cite this article: Williams, I. et al . Direct measurement of osmotic pressure via adaptive confinement of quasi hard disc colloids. Nat. Commun. 4:2555 doi: 10.1038/ncomms3555 (2013).